Optically switchable transistors by simple incorporation of photochromic systems into small-molecule semiconducting matrices The fabrication of multifunctional high-performance organic thin-film transistors as key elements in future logic circuits is a major research challenge. Here we demonstrate that a photoresponsive bi-functional field-effect transistor with carrier mobilities exceeding 0.2 cm 2 V −1 s −1 can be developed by incorporating photochromic molecules into an organic semiconductor matrix via a single-step solution processing deposition of a two components blend. Tuning the interactions between the photochromic diarylethene system and the organic semiconductor is achieved via ad - hoc side functionalization of the diarylethene. Thereby, a large-scale phase-segregation can be avoided and superior miscibility is provided, while retaining optimal π–π stacking to warrant efficient charge transport and to attenuate the effect of photoinduced switching on the extent of current modulation. This leads to enhanced electrical performance of transistors incorporating small conjugated molecules as compared with polymeric semiconductors. These findings are of interest for the development of high-performing optically gated electronic devices. Organic optoelectronic materials [1] attract particular attention for the development of low-cost multifunctional devices, such as phototransistors [2] and optical memories [3] , [4] . In these devices, the light is used as a remote control to modulate electrical properties. In particular, conductivity can be tuned by incorporating photochromic molecules [5] that are able to undergo a reversible light-induced interconversion between the two (or more) isomers possessing markedly different physical and chemical properties [6] , such as different ionization potentials. These different switching states should be thermally stable, and the photoisomerization process should be efficient and highly robust, that is, fatigue resistant. All of these criteria are met by diarylethenes (DAEs) [7] , [8] , which are among the most interesting photochromic molecules to be embedded into thin-film transistors (TFTs) as a single semiconducting component [9] . However, thin films made solely from DAEs suffer from rather poor charge transport properties. This problem can be solved by blending the DAE with organic (semi)conductors such as carbon nanotubes [10] , pentacene [11] or poly(3-hexylthiophene) (P3HT) [12] to combine the light-responsive nature of the DAE with the advantageous charge transport characteristics of the respective matrix component. We have recently shown that by blending DAE and P3HT in solution-processed bi-component films, the P3HT forms polycrystalline structures, while the DAE is dispersed in the less aggregated regions of the polymer film [12] . The good current photoresponse in the TFT can be ascribed to the capacity to introduce within the semiconducting film phototunable and bistable energy levels for the P3HT’s hole transport. Such a blending approach therefore offers a remote control of the output drain current in an organic TFT operated by the light stimuli at defined wavelengths. Our seminal work on blending the DAE with a polymer [12] raised the question of whether such an approach is general and also applicable to small semiconducting molecules. These latter systems typically perform better than semiconducting polymers owing to their enhanced crystallinity, although they may have a stronger tendency to undergo phase segregation when mixed with the DAE molecules. Here we explore the effect of supramolecular organization mediated by the specific substitution pattern of the DAE ( tert -butyl versus methyl) on its photoswitching behaviour when incorporated in both polymeric, as well as small-molecule matrices. On the one hand, P3HT (chemical structure represented in Fig. 1a ) is a model polymeric semiconductor, which is chosen for comparison with our previous study involving DAEs [12] . On the other hand, 2,7-dialkyl-benzothieno(3,2-b)benzothiophene (BTBT) decorated with C 12 H 25 alkyl chains (C 12 BTBT; Fig. 1b ) is selected as the small-molecule semiconducting matrix. Alkyl-substituted BTBT derivatives are particularly suitable as solution-processable, air-stable organic semiconductors, since they possess an extended aromatic core and long aliphatic chains rendering them soluble in common organic solvents. Their solution-processed films showed average mobility values as high as 0.1 cm 2 V −1 s −1 for samples prepared by simple spin-coating [13] , 0.9 cm 2 V −1 s −1 when using a method based on the modified capillary force lithography [14] and 25 cm 2 V −1 s −1 when a novel off-centre spin-coating method is employed [15] . On the other hand, inkjet printing single crystals yielded TFTs for which average mobilities of 16.4 cm 2 V −1 s −1 were reported [16] , whereas 5 cm 2 V −1 s −1 was measured on devices prepared by drop casting on inclined substrates [17] . These values testify that BTBT is among the best performing p-type materials for TFTs, thus competing with their amorphous silicon-based counterparts. As the photochromic component we have selected two DAEs possessing markedly different alkyl substituents, that is, DAE_Me ( Fig. 1c ) and DAE_tBu ( Fig. 1d ). DAE_tBu, with four bulky tert -butyl substituents, is expected to have a much lower propensity to aggregate or interact at the supramolecular level with other alkyl-substituted components, that is, BTBT or P3HT, as compared with DAE_Me carrying only two small methyl groups. 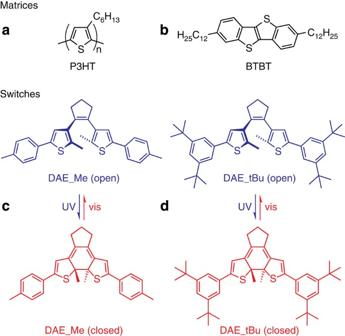Figure 1: Chemical structures of investigated molecules. (a) Polymeric and (b) small molecule semiconducting matrices. (c,d) Photochromic components. Figure 1: Chemical structures of investigated molecules. ( a ) Polymeric and ( b ) small molecule semiconducting matrices. ( c , d ) Photochromic components. Full size image Our results show that small-molecule semiconductors can indeed out-perform their polymeric counterparts in photoresponsive electrical performance when blended with DAE photochromic molecule in TFTs. Both DAE substitution pattern, which controls thin-film morphology, and irradiation conditions, which need to maintain reversibility, turns out to be critical parameters for optimization. Characteristics in the dark We first explore the devices incorporating DAE derivatives in their open form, in the absence of any type of irradiation. The amount of DAEs added to either P3HT or BTBT is 20 wt%. A comparison between the output characteristics ( I D - V D ) of bottom-gate top-contact (BG-TC) devices based on pristine BTBT, as well as BTBT blends with the open forms of DAE_Me and DAE_tBu ( Fig. 2a–c ) shows that they display typical p-type characteristics with a good ohmic contact between BTBT and Au electrodes despite the small injection barrier. These I D - V D curves ( Fig. 2a–c ) also show a good linear and saturation behaviour except for the blend with DAE_Me (open isomer; Fig. 2b ), which exhibits drain current curves that are not completely saturated. From the corresponding transfer characteristics ( I D - V G ) ( Fig. 2e–g ) the relevant device performance in terms of field-effect mobility, threshold voltage and on–off ratio ( I on / I off ) is determined ( Table 1 ). These extracted data reveal that the electronic properties of BTBT are mildly affected by the presence of DAE_tBu in its open form unlike DAE_Me, which drastically decreases the field-effect mobility by two orders of magnitude as compared with the reference device (that is, pristine BTBT). This observation is independent of the device channel length (see Supplementary Fig. 1 ). This finding is in striking contrast with the results obtained on blending of both DAEs (in their open form) with P3HT. In the latter cases, blending P3HT with DAE_Me and DAE_tBu, similar device characteristics as in the reference pristine P3HT are measured as revealed in the output ( Fig. 2d ) and transfer characteristics ( Fig. 2h ), as well as in Table 1 (see also Supplementary Table 1 and Supplementary Fig. 2 ). These results are in line with our previous report on blends of DAE_Me with P3HT, and are explained by the fact that the HOMO (Highest Occupied Molecular Orbital) position of the open form is not accessible for holes, and thus does not affect the charge transport [12] . This is also the case for DAE_tBu bearing a similar HOMO energy level as DAE_Me (see Fig. 3 ). Similar to DAE_Me, it is possible that DAE_tBu does not interfere with the polycrystalline domains but locates in the amorphous regions of P3HT. Moreover, previous reports on combining another DAE derivative with a small molecule, such as pentacene, showed that the HOMO level of the ring-open isomer did not act as a trap level [11] , which is in agreement with our results for P3HT with DAEs. However, for BTBT, the scenario is different since its HOMO level is lying close to the HOMO level of both DAEs in their open form, which renders them accessible for holes (see Fig. 3 ). When DAEs are in their open form, π-conjugation is partially lost and intuitively one would expect a decrease of the device performance owing to the fraction of photochromic molecules, which reduce the number of percolation pathways for charges across the film [9] , [18] . This might explain the poorer electrical characteristics of BTBT devices on addition of the DAE molecules in their open form; but does not account for the large difference observed between the results obtained for the blends with DAE_Me and DAE_tBu, considering that they have similar HOMO energy levels. Furthermore, the threshold voltage of the BTBT devices increases (negatively) on blending with DAE_Me, which is indicative of more disorder, while blending with DAE_tBu leads to only a small variation. The markedly different electrical characteristics in the blends of BTBT with DAE_Me and DAE_tBu (as high as two orders of magnitude in mobility) are rather due to their different morphology: the inclusion of DAE_Me in BTBT domains affects the crystallinity of the latter, ultimately reducing the device dark performance (but not necessarily its photoresponse as will be shown further). 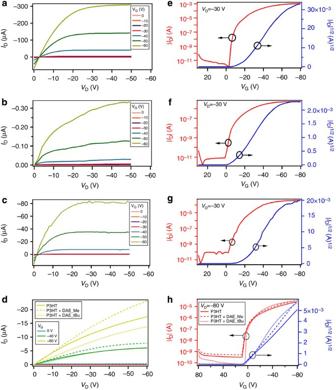Figure 2: Device performance in the dark. Output characteristics of bottom-gate top-contact devices based on (a) pristine BTBT (L=100 μm), (b) BTBT blend with DAE_Me (L=120 μm) and (c) BTBT blend with DAE_tBu (L=120 μm) along with their transfer characteristics (atVD=−30 V) ine,fandg, respectively (left axis in the logarithmic scale; right axis is the square root of the absolute value of the drain current). (d) Output and (h) transfer characteristics of bottom-gate bottom-contact P3HT devices (L=20 μm) blend with DAE_Me, DAE_tBu and without the blend. In this figure, all DAEs are in their open form and mixed with either P3HT or BTBT at 20 wt%. Figure 2: Device performance in the dark. Output characteristics of bottom-gate top-contact devices based on ( a ) pristine BTBT ( L =100 μm), ( b ) BTBT blend with DAE_Me ( L =120 μm) and ( c ) BTBT blend with DAE_tBu ( L =120 μm) along with their transfer characteristics (at V D =−30 V) in e , f and g , respectively (left axis in the logarithmic scale; right axis is the square root of the absolute value of the drain current). ( d ) Output and ( h ) transfer characteristics of bottom-gate bottom-contact P3HT devices ( L =20 μm) blend with DAE_Me, DAE_tBu and without the blend. In this figure, all DAEs are in their open form and mixed with either P3HT or BTBT at 20 wt%. Full size image Table 1 Extracted OFETs parameters from the measurements in dark. 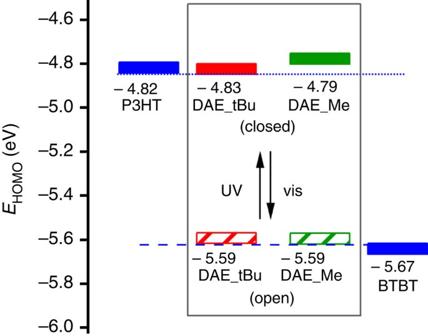Figure 3: Schematic energy level diagram showing the HOMO level of the organic semiconductors used. These values are obtained from cyclic voltammetry. Dotted and dashed lines are guides for the eyes for comparing the HOMO level of P3HT with DAEs in their closed form, and BTBT with DAEs in their open form. DAEs are highlighted in a rectangle and the arrows indicate the change of the energy level on irradiation with either ultraviolet or visible light. Full size table Figure 3: Schematic energy level diagram showing the HOMO level of the organic semiconductors used. These values are obtained from cyclic voltammetry. Dotted and dashed lines are guides for the eyes for comparing the HOMO level of P3HT with DAEs in their closed form, and BTBT with DAEs in their open form. DAEs are highlighted in a rectangle and the arrows indicate the change of the energy level on irradiation with either ultraviolet or visible light. Full size image Initial miscibility studies conducted by differential scanning calorimetry did not provide any obvious evidence of phase separation, showing that both DAE_Me and DAE_tBu (open form) are miscible with BTBT. Interestingly, miscibility of BTBT with DAE_Me is found to be higher as compared with DAE_tBu (see Supplementary Figs 3–8 ). To cast further light onto the internal structure of the different blends, we performed grazing incidence X-ray diffraction (GIXD) measurements using synchrotron radiation ( Supplementary Figs 9,10 ). The results show that the BTBT/DAE_tBu blend exhibits a crystalline structure closely resembling that of a pure BTBT film. The diffraction pattern for the BTBT/DAE_Me blend indicates that the texture of the crystallites is altered on blending due to the nucleation of highly misoriented crystallites ( Supplementary Figs 9,10 ). In fact, 33% of the BTBT crystallites in the BTBT/DAE_Me blend lie 70° from the substrate normal such that the insulating alkyl side chains are close to parallel to the film substrate. This markedly affects the charge carrier mobility and significantly lowers the device performance ( Supplementary Fig. 11 ). In stark contrast, no misoriented crystallites are observed in pure BTBT or BTBT/DAE_tBu blend. Notably, AFM measurements on the sub-micrometre scale do not reveal any difference in the morphology of films of P3HT and BTBT when blended with DAE_Me or DAE_tBu ( Supplementary Figs 12–14 ). We can therefore conclude that the perturbation of the BTBT crystals or phase segregation due to the presence of the DAEs is on a length scale below 150 nm. In agreement with the diffraction results, optical spectroscopy studies also suggest a change in the properties of blend films when BTBT is crystallized in the presence of DAE_Me as compared with DAE_tBu. Absorption spectra of the blends ( Supplementary Fig. 15 ) show that the BTBT absorption band at 365 nm is broadened and blue-shifted when blended with DAE_Me, whereas it is mostly unaffected when blended with DAE_tBu (see also Supplementary Figs 16 and 17 for blends with P3HT and for pristine DAEs). Confocal fluorescence imaging of the BTBT/DAE_Me (closed form) blend reveals green emission from areas that correspond exactly to regions of large BTBT crystallites (see Fig. 4a and Supplementary Fig. 18a,c ), whereas for both the BTBT/DAE_tBu (closed isomer) blend and neat BTBT films only homogeneous emission is observed across the field of view at the same wavelengths. Identifying the exact origin of the absorption broadening and green emission is beyond the scope of this work, but nevertheless confirms the markedly different optical properties of the BTBT/DAE_Me and BTBT/DAE_tBu blends. Only in case of the BTBT/DAE_tBu (closed form) blend, red emission is observed from localized crystallites (see Fig. 4b and Supplementary Fig. 18b,d ), spectrally similar to the emission of neat films of the DAEs in their closed form (see Supplementary Fig. 19 ). The fact that no such red emission is observed from the BTBT/DAE_Me (closed isomer) films strengthens the assertion that DAE_Me (closed isomer) associates more strongly with BTBT compared with DAE_tBu (closed isomer) due to steric factors caused by the tert -butyl substituents. Note that there is no difference in the emission properties of the P3HT blends with DAE_Me and DAE_tBu. 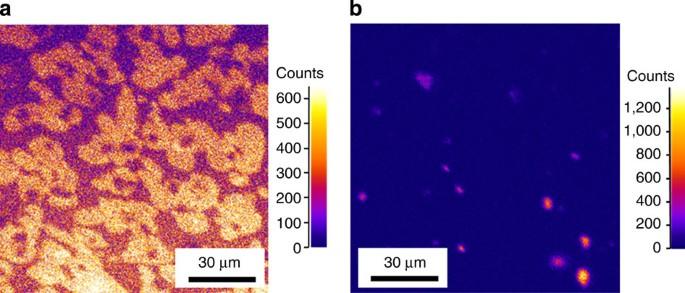Figure 4: Emission in blend films. Scanning confocal fluorescence microscopy images (excitation at 405 nm) revealing the emission of films of: (a) BTBT blend with DAE_Me (at 530±15 nm) and (b) BTBT blend with DAE_tBu (at 605±35 nm). Figure 4: Emission in blend films. Scanning confocal fluorescence microscopy images (excitation at 405 nm) revealing the emission of films of: ( a ) BTBT blend with DAE_Me (at 530±15 nm) and ( b ) BTBT blend with DAE_tBu (at 605±35 nm). Full size image Photoswitching Next, we investigate the switching characteristics of the corresponding BG-TC devices on illumination with the light of different wavelengths ( Fig. 5 ). Note that bottom-gate bottom-contact (BG-BC) devices have also been studied (see Supplementary Figs 20–22 and Supplementary Note 2 ). Starting with the P3HT blends, on initial exposure to successive illumination of ultraviolet light ( λ =365 nm) divided into three steps of 90 s, 2 min and 10 min, the maximum of the normalized drain current at fixed gate ( V G =−80 V) and drain biases ( V D =−10 V) decreases consecutively at each step and reaches a maximum loss of 68% for the P3HT/DAE_Me blend and 22% for the P3HT/DAE_tBu blend ( Fig. 5a ). Clearly, ultraviolet irradiation induces photochemical conversion of the open to the closed DAE isomers. As a consequence, the energy difference (ΔΦ) between the HOMO levels of the host and guest molecules is now an intragap level for the holes transported in the semiconducting layer ( Fig. 3 ); once there, the charges are trapped at the closed switch [11] . In view of the very similar HOMO energy levels of the two DAE derivatives in their closed form, the observed large difference in current modulation seems to be the result of their very different interaction with P3HT. On irradiation with visible light ( λ =546 nm for 12 min in total), a reversible change in the drain current was obtained and the initial characteristics of the devices were regained progressively for both P3HT films with DAE_Me and DAE_tBu due to the photochemical ring opening of the closed DAEs back to their open forms. The photoswitching behaviour was reproducible for additional cycles, alternating between ultraviolet and visible light irradiations. Note that BG-BC devices show comparable current modulation trends under illumination ( Supplementary Fig. 20 ) as compared with the BG-TC devices and similar to those reported for P3HT with DAE_Me. 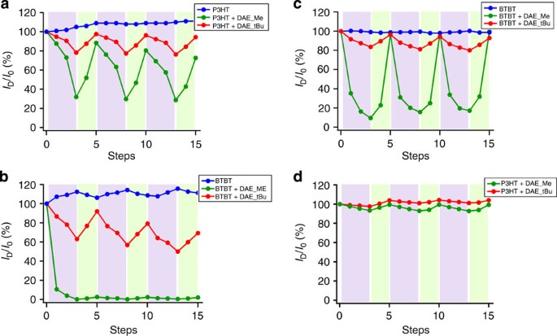Figure 5: Repeated switching cycles. The normalized maximum drain current extracted from the transfer characteristics at fixed gate (VG=−80 V) and drain biases (VD=−10 V) is plotted in function of the irradiation sequence. Comparison between the photoswitching of (a) P3HT-based TFTs and (b) BTBT-based devices for long ultraviolet irradiation time. (candd) Comparison of the photoswitching of BTBT- and P3HT-based TFTs, respectively, for a short ultraviolet irradiation time. In all the graphs, light violet and light green shaded areas correspond to the irradiation with light at wavelengths of 365 and 546 nm, respectively. All the devices irradiated feature BG-TC geometry. [12] Figure 5: Repeated switching cycles. The normalized maximum drain current extracted from the transfer characteristics at fixed gate ( V G =−80 V) and drain biases ( V D =−10 V) is plotted in function of the irradiation sequence. Comparison between the photoswitching of ( a ) P3HT-based TFTs and ( b ) BTBT-based devices for long ultraviolet irradiation time. ( c and d ) Comparison of the photoswitching of BTBT- and P3HT-based TFTs, respectively, for a short ultraviolet irradiation time. In all the graphs, light violet and light green shaded areas correspond to the irradiation with light at wavelengths of 365 and 546 nm, respectively. All the devices irradiated feature BG-TC geometry. Full size image In the BTBT blends with DAE_tBu and DAE_Me, over the same, long ultraviolet illumination times, the current decreases for each step and it is lowered by 40% and almost 100%, respectively, at step 3 ( Fig. 5b ). This is indicative of deeper traps for holes due to higher ΔΦ with BTBT as compared with P3HT. Therefore, DAEs in their closed form act as shallow traps with P3HT but as deep traps with BTBT in agreement with predictions for F8BT [19] . Comparing both DAEs, the trend in the current variation is similar to the one for the blends with P3HT but with greater modulation. Surprisingly, on irradiation with visible light, the drain current is recovered only in the case of DAE_tBu (although with a gradual decrease over repeated switching cycles), while no recovery is observed for the BTBT/DAE_Me blend ( Fig. 5b and Supplementary Fig. 23 ). The observed irreversibility could be the result of a strong association of DAE_Me (closed form) with the network of BTBT crystallites, thereby suppressing photoswitching of DAE_Me back into its open form. Similar phenomena have been observed previously where it was shown that the photochromism of DAEs is strongly dependent on their environment and arrangement in the solid [20] , [21] , [22] . An alternative explanation may be given considering the photochemically induced degradation of the DAEs, which on prolonged ultraviolet irradiation forms a by-product [23] (see below). In the absence of the DAE derivatives, both matrices, that is, pristine P3HT and BTBT, exhibit a small increase of the drain current during irradiation with either ultraviolet or visible light ( Fig. 5a,b ; blue plots) originating from photogenerated carriers. Noteworthy, it appears that no ring closure due to current flow is occurring in bi-component films, in contrast to previous observations on neat films of photochromic moieties in vertical geometries [4] , [24] . This is supported by comparing single- and bi-component film devices (see Supplementary Fig. 20b ) and further confirmed by the fact that our devices include no neat films of DAEs, and therefore the current passes primarily through the crystalline portions of the semiconductor film; a planar geometry is employed in which the transversal electric field ( V DS / L ) is generally lower than in vertical geometries; no decrease in current was observed on operating bi-component devices in the dark, indicating the absence of traps and hence current-induced formation of ring-closed DAE isomers. To gain further insight into the photoswitching of DAE and particularly its irreversibility for DAE_Me blends with BTBT on elongated ultraviolet irradiation times, we determine the isomerization quantum yield for the conversion of the closed to the open form in films of BTBT and P3HT ( Supplementary Table 3 ). We found that the isomerization quantum yield in the films is lower than in solution but still high enough for all blends to impose no practical problem of photoswitching in the TFT device. The quantum yield is higher in P3HT as compared with BTBT for both the DAE derivatives and higher in the presence of the tert -butyl group in DAE_tBu as compared with DAE_Me (see Supplementary Table 3 ). However, in view of the unexpected behaviour of BTBT/DAE_Me and to regain the initial device characteristics on irradiation with the visible light, we limit the ultraviolet irradiation time to a maximum of 30 s (in three steps of 10 s each). The same irradiation procedure is followed on irradiation with visible light. Gratifyingly, BTBT/DAE_Me shows a reproducible and large (maximum variation up to 90%) modulation of the drain current ( Fig. 5c ), whereas BTBT/DAE_tBu reveals only a small drain current modulation (by 20%). In contrast to the BTBT blended devices, the current modulation for P3HT blends is very low (<10% for DAE_Me and 3% for DAE_tBu with P3HT, Fig. 5d ) at this short ultraviolet irradiation time (see also Supplementary Fig. 24 ). Since the large difference in photomodulation efficiency between the two DAEs cannot be explained purely by energetics, the open to closed isomerization in BTBT blends is examined using ultraviolet–visible spectroscopy. For BTBT/DAE_tBu blends, the logarithmic absorbance as a function of irradiation time followed a linear dependence ( Supplementary Figs 26, 28,29 and Supplementary Note 3 ). However, for the BTBT/DAE_Me blends, systematic deviations from linearity can be observed: at short timescales a faster rate of conversion can be monitored than on longer timescales ( Supplementary Fig. 29 ). This more complex behaviour of the isomerization kinetics of the BTBT/DAE_Me blend indicates that DAE_Me experiences (at least) two different environments in the films: likely a restricted one corresponding to more crystalline areas of the film and another one corresponding to less aggregated portions of the film, as confirmed by GIXD, with much reduced intermolecular interactions. We note that while the kinetic analysis does not take the possible effects of by-product formation into account, the results fit perfectly with the XRD and optical data. Thus, the higher modulation amplitude of BTBT/DAE_Me devices can be explained by the higher proportion of DAE_Me molecules blended in the BTBT matrix where their photoisomerization should have the greatest effect on percolation pathways. Thus, on short ultraviolet irradiation times, the isomerization of a small fraction of the DAE molecules in the BTBT/DAE_Me blend is sufficient to induce a large effect on the current output of the device. A possible explanation for the observed irreversibility of the current modulation in the BTBT/DAE_Me device on prolonged ultraviolet irradiation involves the formation of a small amount of by-product present after the initial ring-closing step. Given the similar π-electronic structure of the closed isomer and the by-product [23] , the latter should also be able to act as a trap within the semiconductor blend. Although the fatigue behavior of both DAE_Me and DAE_tBu should be rather similar, as demonstrated by repetitive switching cycles in solution (see Supplementary Fig. 27 ), the formation of the by-product as a trap seems to have a much more pronounced effect on the (irreversible) current modulation in the case of the BTBT/DAE_Me device. This is in analogy to the finding that during short ultraviolet irradiation only a small fraction of the DAE_Me molecules ring-close, and hence only few trapping sites are sufficient to efficiently obstruct current flow through the device (due to the strong association between DAE_Me and BTBT). In contrast, a higher conversion to the ring-closed isomer producing a larger amount of trapping sites is necessary to achieve the same current modulation in the case of DAE_tBu. Thus, only after several switching cycles, an increasing amount of formed by-product decreases the overall switching efficiency of the BTBT/DAE_tBu device. In view of all the above results, it is clear that photoresponsive TFT performance is the result of a complex interplay of supramolecular photochrome–matrix interactions, their effect on charge transport on the one hand and photoswitching ability as well as photoreversibility on the other hand, and hence the applied irradiation conditions. Considering the bulky DAE_tBu having weaker interactions with the hosting matrix, both the dark performance and the photomodulation are superior for the small-molecule semiconductor BTBT blend versus the polymeric semiconductor P3HT blend. However, if strong photomodulation is a priority, DAE_Me is the preferred photochrome reaching modulations of up to 90% for the BTBT blend, but at the price of reduced dark performance and increased sensitivity towards photodegradation after prolonged ultraviolet light exposure. In summary, we extend our approach of blending photochromic systems with a polymer to small molecules, which are known to exhibit greater device performance when integrated in TFTs. Ad-hoc molecular design made it possible to control the interactions between the two components, and thus the structure/morphology within the films along with their respective energy levels, ultimately affecting the charge transport in the device, as well as the current photomodulation, and hence, the overall switching performance. In particular, by phototuning the energy level in a bi-component organic semiconductor, we study the effect of photochromic molecules with different alkyl substituents on the electrical performance of TFTs based on P3HT and BTBT. By exploiting the exceptional electronic characteristics of BTBT, we are able to fabricate optically switchable transistors with charge carrier mobilities as high as 0.21 cm 2 V −1 s −1 . Interestingly, the properly designed DAE_tBu revealed very mild alteration of the BTBT structure within the blend films, which is reflected by almost unaffected device performance in dark conditions while maintaining good (40%) photomodulation. Alternatively, photomodulation can be increased to 90% by employing DAE_Me; however, this changes the structure of the BTBT matrix, reducing its dark performance. The above results prove that our blending approach is generally applicable to organic semiconducting molecules and can be tuned to fit the priority function of the device in question. These findings are attractive for the development of high-performing optically gated electronic devices for potential applications in memories, logic circuits and more generally in optoelectronics and optical sensing. General remarks The syntheses of BTBT and DAE_Me are carried out according to the published procedures [12] , [13] , [25] . For synthesis and characterization of tert -butyl-substituted DAE_tBu see the Supplementary Figs 32–33 and Supplementary Method . Photochromic properties of pristine DAEs are reported in Supplementary Table 2 and their absorption spectra are reported in Supplementary Fig. 25 . Composition and preparation of the blends DAE_Me and DAE_tBu are blended with BTBT or P3HT. The composition of DAE is always 20 wt% (this percentage is chosen for comparison with our previous work [12] ). Blends are fabricated by mixing compounds in chloroform. The final concentration of BTBT in the blend is 4 mg ml −1 and for P3HT is 1 mg ml −1 . These solutions were subsequently spin coated. Device fabrication BG-TC transistors are fabricated on heavily doped n-type silicon wafers serving as gate electrode with 230-nm thick thermally grown SiO 2 as the dielectric layer ( C i =15 nF cm −2 ). These substrates are ultrasonically cleaned with acetone and isopropanol, and then dried with nitrogen. The surface of the dielectric is treated with ozone (three cycles consisting each of 5-min ozone generation followed by 25-min incubation) and then the devices are transferred to the glovebox. As for the semiconducting layer, first we prepare solutions composed of blends of DAE_Me or DAE_tBu (in their open form) with P3HT or BTBT as above mentioned. These solutions are deposited by spin-coating at 3500, r.p.m. for 30 s followed by thermal annealing at 80 °C for 30 min as per the procedure we recently reported [26] for the case of solutions containing BTBT. As for solutions containing P3HT, they are spin coated at 1500, r.p.m. for 60 s. Right after, top Au source and drain electrodes are evaporated using a shadow mask (thickness=35 nm, chamber pressure=10 −6 mbar, evaporation rate=0.03 nm s −1 ) with different channel length ( L =60, 80, 100 and 120 μm) and constant channel width ( W =10 mm). For comparison, reference devices based on pristine BTBT (4 mg ml −1 ) and P3HT (1 mg ml −1 ) are prepared in the same manner. Also BG-BC devices based only on the blends with P3HT are fabricated for comparison with the previous work on DAE_Me [12] . They feature pre-patterned interdigitated electrodes (with L =20 μm and W =10 mm) with the same specifications as above mentioned. The fabrication of BG-BC FETs with BTBT has been explored yet yielded non-functioning devices [26] . Electrical characterization Electrical characterization of the devices is performed at room temperature in a N 2 atmosphere inside a glovebox, using a Cascade Microtech M150 probe station and a Keithley 2636A controlled by Labtracer software. Field-effect mobility and threshold voltage are extracted from the saturation regime at V D =−30 V. See also Supplementary Note 1 . Irradiation procedure for the static switching Three cycles are performed consisting each of: Step 0 in the dark. Steps 1, 2 and 3: irradiation with λ =365 nm for 90 s, additional 120 s and additional 600 s, respectively. This is followed by 300 s of relaxation under dark. Steps 4 and 5: irradiation with λ =546 nm for 120 s and additional 600 s, respectively. For all the steps after irradiation, the light is switched off and the value of the drain current at V D =−10 V and V G =−80 V is taken from the full I D - V G curve. We also performed another procedure by limiting the irradiation in the ultraviolet to 10 s for each step and keeping the same irradiation time at λ =546 nm. Instrumentation Devices are irradiated from the top using a Polychrome V (Till Photonics) tunable light source providing a monochromatic beam with λ =365 and 546 nm with irradiance levels of 0.6 and 13.94 mW cm −2 , respectively. The light intensity is measured using an analogue optical power metre, PM100A (ThorLabs). The wavelengths are chosen in accordance to our previous study to facilitate a comparison. Ultraviolet–visible spectra are recorded on JASCO V-670 spectrophotometer. For both the DAE derivatives, the HOMO levels are determined by cyclic voltammetry CV (see Supplementary Figs 30,31 , Supplementary Table 4 , Supplementary Note 4 and Supplementary Method ). For comparison, also HOMO levels of BTBT and P3HT are determined by CV. Two-dimensional GIXD with a MAR345 image plate is performed on beam line 11-3 at the Stanford Synchrotron Radiation Light source with an incident energy of 12.7 keV. The measurements are collected at a grazing angle of 0.1° and expressed as a function of the scattering vector q =4 π sin( θ )/ λ . Here θ represents half of the scattering angle, λ is the wavelength of the incident beam, q xy is the component of the scattering vector parallel to the substrate plane and q z is the component perpendicular to the substrate plane. Atomic force microscopy (AFM) images are recorded in tapping mode using a Nanoscope (Veeco Multimode V) on the same devices characterized. Fluorescence images are acquired with a Nikon Eclipse Ti scanning confocal fluorescence microscope, using continuous wave excitation at 405 nm. A × 60 magnification, 0.95 numerical aperture plan apo air objective, a 100-μm diameter confocal pinhole, a 515±15 and 605±35 nm band-pass filters before the detector. Fluorescence images are recorded after the samples were irradiated with a ultraviolet lamp at 365 nm for 2 min to trigger the isomerization of DAE molecules from the open to the closed form. How to cite this article : Gemayel, M. E. et al . Optically switchable transistors by simple incorporation of photochromic systems into small-molecule semiconducting matrices. Nat. Commun. 6:6330 doi: 10.1038/ncomms7330 (2015).